Receptor tyrosine kinase ErbB2 translocates into mitochondria and regulates cellular metabolism It is well known that ErbB2, a receptor tyrosine kinase, localizes to the plasma membrane. Here we describe a novel observation that ErbB2 also localizes in mitochondria of cancer cells and patient samples. We found that ErbB2 translocates into mitochondria through association with mtHSP70. Additionally, mitochondrial ErbB2 (mtErbB2) negatively regulates mitochondrial respiratory functions. Oxygen consumption and activities of complexes of the mitochondrial electron transport chain were decreased in mtErbB2-overexpressing cells. Mitochondrial membrane potential and cellular ATP levels were also decreased. In contrast, mtErbB2 enhanced cellular glycolysis. The translocation of ErbB2 and its impact on mitochondrial function are kinase dependent. Interestingly, cancer cells with higher levels of mtErbB2 were more resistant to the ErbB2-targeting antibody trastuzumab. Our study provides a novel perspective on the metabolic regulatory function of ErbB2 and reveals that mtErbB2 has an important role in the regulation of cellular metabolism and cancer cell resistance to therapeutics. Most cancer cells take up glucose at higher rates than normal cells, but use a smaller fraction of this glucose for oxidative phosphorylation [1] , [2] , [3] , [4] , [5] , [6] , [7] , [8] , [9] . Although the molecular mechanisms underlying this phenomenon remain unclear, increased glycolysis in cancer cells has been well accepted to be an important process to support malignant phenotypes [6] . The importance of this effect is further underscored by recent studies, which reported that impaired mitochondrial function renders cancer cells resistant to apoptosis and chemotherapy [10] , [11] . Our recent studies also demonstrated that inhibiting glycolysis sensitizes cancer cells to the chemotherapeutic agent paclitaxel [12] and ErbB2-targeting antibody trastuzumab [13] . This suggests that mitochondrial function and cellular metabolism have a critical role in cancer progression and therapeutic resistance. ErbB2 (also known as Her2/neu) is an oncogene that is overexpressed in many types of cancers and is correlated with a poor prognosis [14] . We and others [15] , [16] , [17] , [18] , [19] have previously demonstrated that ErbB2 increases the transformation and/or metastatic potential of human breast cancer. In addition, ErbB2 has been shown to activate signalling molecules which regulate bioenergetic metabolism [17] , [19] , [20] , [21] , [22] . Our previous study showed that ErbB2 promotes cancer cell growth and glycolysis through increased expression of lactate dehydrogenase isoform A (LDH-A) [23] . However, it is unclear whether, in addition to the enhancement of glycolysis, ErbB2 also regulates cell metabolism through additional processes. It is well established that ErbB2 localizes to the plasma membrane where it phosphorylates downstream substrates on their tyrosine residues in response to extracellular stimulation. Recent studies also have shown that ErbB2 can translocate into the nucleus and putatively function as a transcription factor [24] . One study has shown that Heregulin β1 regulates cytochrome c oxidase subunit II in mammary epithelial cells [25] . Another report described that the blockade of the ErbB2 receptor induces cardiomyocyte death through mitochondria and reactive oxygen species-dependent pathways [26] . Moreover, tyrosine phosphorylation and de-phosphorylation of proteins in mitochondria have been reported through several important kinases and phosphatases, such as PKC and Abl [27] , Src [28] , MAPK [29] and Shp-2 (ref. 30 ). In addition, EGFR, another member of the EGFR family proteins has been reported to translocate into mitochondria [31] . These studies suggest that the subcellular localization of ErbB2 may define its signalling specificity and ErbB2 may regulate mitochondrial functions. Localization of ErbB2 in mitochondria of cancer cells While investigating the role of ErbB2 in regulating cellular metabolism, we unexpectedly observed that ErbB2 also exists in the mitochondria of ErbB2-positive breast cancer cells. We analysed the organelle fractions from multiple breast cancer cell lines and patient samples ( Supplementary Methods ). In addition to plasma membrane and cytoplasmic fractions, ErbB2 was present in mitochondrial fraction of two ErbB2-transfected cancer cell lines MCF7/ErbB2 and MDA-MB-231/ErbB2, and of two natural ErbB2-positive cancer cell lines BT474 and SKBR3, detected by western blotting ( Fig. 1a ). To eliminate the possibility that the bands of mtErbB2 were due to contamination from other organelles, the western blots were probed for different cellular organelle markers. The results indicate that the mitochondrial fraction we prepared was of high purity. Similar results were obtained from tumour samples of ErbB2-positive breast cancer patients and the MCF7 breast cancer cells, which express moderate levels of ErbB2 ( Fig. 1b ). We also observed that ErbB2 also localized in the mitochondria of the heart and liver tissues of normal mouse ( Fig. 1b ), suggesting that the mitochondrial localization of ErbB2 is not due to overexpression of ErbB2, which may lead to mislocalization. 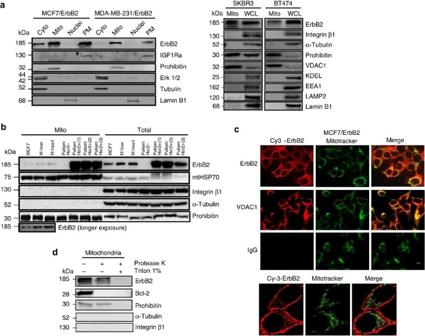Figure 1: Localization of ErbB2 in mitochondria. (a) Cytosolic, nuclear, mitochondrial and plasma membrane proteins were isolated and subjected to SDS–PAGE followed by probing with indicated antibodies. Two exogenous ErbB2 overexpressing breast cancer cell lines MCF7/ErbB2 and MDA-MB-231/ErbB2 (left), and two natural ErbB2-positive breast cancer cell lines SKBR3 and BT474 (right) were used for western blotting. VDAC1 and prohibitin were mitochondrial markers; Integrin β1 and IGF1Rα were plasma membrane markers; α-tubulin and ERK were cytoplasmic markers; KDEL was an ER marker; EEA1 was an early endosomes marker; LAMP2 was an lysosome marker and Lamin B1 was a nucleus marker. (b) MCF7 cells, mouse heart and liver tissues, and ErbB2-positive and -negative breast cancer patient samples were analysed by western blotting. (c) Co-localization of ErbB2 and mitochondria. Mitochondria were stained with Mitotracker-Green in ErbB2-transfected MCF7 cells. The cells were fixed and incubated with antibodies against ErbB2 (mouse), followed by incubation of monoclonal mouse anti-Cy3 antibody (red). Images were analysed with Nikon NIS-Elements AR software. Green, mitochondria; red, ErbB2; yellow, co-localization of ErbB2 and mitochondria. The lower panel contains images with a higher magnification. Scale bars, 20 μm. (d) Localization of ErbB2 inside mitochondria. Intact mitochondria of SKBR3 cells were isolated and treated with Protease K at 0.5 mg ml−1for 15 min at room temperature. 1% Triton was added into the reaction and 2 mM PMSF was added to stop the reaction. Each reaction was started with an equal amount per volume of mitochondria lysate. Mitochondrial lysate then was loaded onto 8% SDS–PAGE followed by blotting with anti-ErbB2, anti-BCL-2 and anti-prohibitin antibodies. Figure 1: Localization of ErbB2 in mitochondria. ( a ) Cytosolic, nuclear, mitochondrial and plasma membrane proteins were isolated and subjected to SDS–PAGE followed by probing with indicated antibodies. Two exogenous ErbB2 overexpressing breast cancer cell lines MCF7/ErbB2 and MDA-MB-231/ErbB2 (left), and two natural ErbB2-positive breast cancer cell lines SKBR3 and BT474 (right) were used for western blotting. VDAC1 and prohibitin were mitochondrial markers; Integrin β1 and IGF1Rα were plasma membrane markers; α-tubulin and ERK were cytoplasmic markers; KDEL was an ER marker; EEA1 was an early endosomes marker; LAMP2 was an lysosome marker and Lamin B1 was a nucleus marker. ( b ) MCF7 cells, mouse heart and liver tissues, and ErbB2-positive and -negative breast cancer patient samples were analysed by western blotting. ( c ) Co-localization of ErbB2 and mitochondria. Mitochondria were stained with Mitotracker-Green in ErbB2-transfected MCF7 cells. The cells were fixed and incubated with antibodies against ErbB2 (mouse), followed by incubation of monoclonal mouse anti-Cy3 antibody (red). Images were analysed with Nikon NIS-Elements AR software. Green, mitochondria; red, ErbB2; yellow, co-localization of ErbB2 and mitochondria. The lower panel contains images with a higher magnification. Scale bars, 20 μm. ( d ) Localization of ErbB2 inside mitochondria. Intact mitochondria of SKBR3 cells were isolated and treated with Protease K at 0.5 mg ml −1 for 15 min at room temperature. 1% Triton was added into the reaction and 2 mM PMSF was added to stop the reaction. Each reaction was started with an equal amount per volume of mitochondria lysate. Mitochondrial lysate then was loaded onto 8% SDS–PAGE followed by blotting with anti-ErbB2, anti-BCL-2 and anti-prohibitin antibodies. Full size image To further verify these results, fluorescent microscopy was performed using the MCF7/ErbB2 cells. The images showed that ErbB2 (red) was sporadically distributed in the cytoplasm in addition to the strong staining of the plasma membrane ( Fig. 1c ). After merging red (ErbB2) and green (Mitotracker), the image showed a yellow colour, supporting that ErbB2 is present in mitochondria. Similar results were also detected in SKBR3 cells, which naturally overexpress endogenous ErbB2 ( Supplementary Fig. S1 ). The mitochondrial localization of ErbB2 was further confirmed by immuno-gold transmission electron microscopy in SKBR3 cells ( Supplementary Fig. S2 ). To determine whether ErbB2 was inside of mitochondria, we conducted protease sensitivity experiments by incubation of mitochondria with proteinase K in the presence or absence of Triton-X100. Without Triton-X100, ErbB2 and prohibitin (an inner membrane protein) were resistant to proteinase K, whereas Bcl-2, which is localized on the outer membrane, was degraded ( Fig. 1d ). When proteinase K was added to mitochondria in the presence of Triton-X100, all of the proteins were degraded, indicating that like prohibitin, ErbB2 exists inside of mitochondria. Identification of the mitochondrial-targeting sequence (MTS) We next studied whether ErbB2 has an endogenous MTS and how ErbB2 translocates into mitochondria. An online mitochondrial localization prediction program showed that ErbB2 has a strong possibility of localizing in mitochondria ( Supplementary Table S1 ), suggesting that ErbB2 may have an endogenous MTS. The juxtamembrane region of the ErbB2 contains basic amino acids, which are similar to other known mitochondrial proteins, such as Tom20. These proteins contain a MTS consisting of highly hydrophobic and basic amino-acid-rich sequences in their transmembrane domains (TMD) and membrane-flanking regions. To determine whether the juxtamembrane region of ErbB2 constitutes a functional MTS, expression plasmids encoding GFP-tagged ErbB2 trans- and juxtamembrane sequences were constructed ( Fig. 2a ). The constructs included GFP alone, GFP plus the ErbB2 juxtamembrane region (aa 646–689), GFP fused with TMD (aa 623–645), and GFP plus TMD fused with juxtamembrane region (aa 623–689). These constructs were transfected into MCF7 cells. The location of GFP alone and the GFP-ErbB2 fusion proteins was determined by fluorescent microscopy. The results showed that the juxtamembrane (aa 646–689) domain contains a nuclear localization signal and the distribution of GFP was mostly in the nucleus. TMD alone (aa 623–645) was insufficient to target GFP into mitochondria. However, the fused domains (aa 623–689) did target the GFP into mitochondria, indicating that this region is sufficient for ErbB2 localization to the mitochondria. 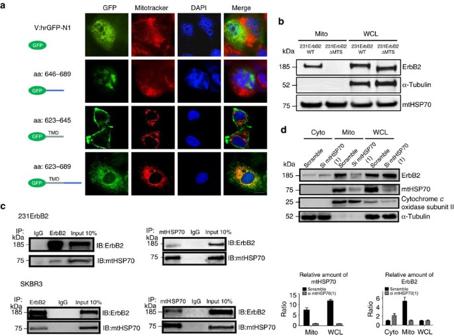Figure 2: Analysis of the mechanisms of mtErbB2 mitochondrial localization. (a) MCF7 breast cancer cells were transfected with plasmids encoding either GFP alone, or GFP-fused ErbB2 fragments GFP-646–689, GFP-623–645 or GFP-623–689. Cells were cultured and the fluorescent imaging was done as described in the Methods. Scale bars, 20 μm. (b) MDA-MB-231 cells were transfected with wild-type ErbB2 and ErbB2ΔMTS vectors and mitochondrial proteins were extracted. ErbB2 expression was measured by western blotting analysis; α-tubulin and mtHSP70 were loading controls. (c) Mitochondrial proteins were isolated from MDA-MB-231/ErbB2 cells and immunoprecipitated with ErbB2 antibody. The immunoprecipitates were probed with anti-mtHSP70 and anti-ErbB2 (top left). Mitochondrial proteins from the same cells were precipitated with mtHSP70 antibody and the immunoprecipitates were probed with anti-mtHSP70 and anti-ErbB2 (top right). IgG was used as a negative control. Isolated mitochondrial proteins (input) were loaded as a positive control. Similar results were obtained using another breast cancer cell line, SKBR3 (bottom). (d) siRNA specific to mtHSP70 was transfected into MDA-MB-231/ErbB2 cells. The cytoplasmic fraction (Cyto), mitochondrial fraction (Mito) and whole-cell lysate (WCL) were separated for western blotting analysis (left). Cytochromecoxidase subunit II and α-tubulin were makers and loading controls for the mitochondrial fraction and the cytoplasmic fraction, respectively. The relative protein amounts of ErbB2 and mtHSP70 were calculated by determining the intensity of the protein bands followed by the normalization with loading controls (right). Experiments were repeated three times. Columns, mean of three independent experiments; bars, s.e. IP, immunopreciptation; IB, immunoblotting. Figure 2: Analysis of the mechanisms of mtErbB2 mitochondrial localization. ( a ) MCF7 breast cancer cells were transfected with plasmids encoding either GFP alone, or GFP-fused ErbB2 fragments GFP-646–689, GFP-623–645 or GFP-623–689. Cells were cultured and the fluorescent imaging was done as described in the Methods. Scale bars, 20 μm. ( b ) MDA-MB-231 cells were transfected with wild-type ErbB2 and ErbB2ΔMTS vectors and mitochondrial proteins were extracted. ErbB2 expression was measured by western blotting analysis; α-tubulin and mtHSP70 were loading controls. ( c ) Mitochondrial proteins were isolated from MDA-MB-231/ErbB2 cells and immunoprecipitated with ErbB2 antibody. The immunoprecipitates were probed with anti-mtHSP70 and anti-ErbB2 (top left). Mitochondrial proteins from the same cells were precipitated with mtHSP70 antibody and the immunoprecipitates were probed with anti-mtHSP70 and anti-ErbB2 (top right). IgG was used as a negative control. Isolated mitochondrial proteins (input) were loaded as a positive control. Similar results were obtained using another breast cancer cell line, SKBR3 (bottom). ( d ) siRNA specific to mtHSP70 was transfected into MDA-MB-231/ErbB2 cells. The cytoplasmic fraction (Cyto), mitochondrial fraction (Mito) and whole-cell lysate (WCL) were separated for western blotting analysis (left). Cytochrome c oxidase subunit II and α-tubulin were makers and loading controls for the mitochondrial fraction and the cytoplasmic fraction, respectively. The relative protein amounts of ErbB2 and mtHSP70 were calculated by determining the intensity of the protein bands followed by the normalization with loading controls (right). Experiments were repeated three times. Columns, mean of three independent experiments; bars, s.e. IP, immunopreciptation; IB, immunoblotting. Full size image To determine whether the basic amino-acid-rich sequence in the juxtamembrane and transmembrane region was required for ErbB2 translocation into mitochondria, expression plasmids encoding ErbB2 with an aa 623–689 deletion (ErbB2ΔMTS) were transfected into MDA-MB-231 cells. The mitochondrial fractions were isolated and the samples subjected to western blotting analysis. Figure 2b shows that ErbB2 with the aa 623–689 deletion could not translocate into mitochondria, defining a novel mitochondrial-targeting function of this region in ErbB2. We also conducted confocal imaging analysis and the co-localization was analysed by NIH ImageJ software in 231ErbB2WT, 231ErbB2Mito and 231ErbB2ΔMTS cells. Approximately 80% 231ErbB2Mito cells showed mitochondrial localization of ErbB2 and only 10% 231ErbB2ΔMTS cells showed mtErbB2 localization (data not shown). Together, these results clearly indicate that the TMD plus aa 646–689 of ErbB2 are both sufficient and necessary for mitochondrial localization of ErbB2. mtHSP70-dependent translocation of ErbB2 To study how ErbB2 was translocated into mitochondria, immunoprecipitation with antibodies against ErbB2 was conducted using mitochondrial proteins extracted from ErbB2-positive SKBR3 cells to identify mitochondrial proteins that interact with ErbB2. An SDS–polyacrylamide gel electrophoresis (SDS–PAGE) gel of the immunoprecipitated proteins was stained with Coomassie Blue. The proteins extracted from the gel were subjected to mass spectrometry. Supplementary Fig. S3 shows that among the candidate proteins that are associated with ErbB2, one protein has a molecular weight of ~70 kDa. This protein was identified as mtHSP70 by mass spectrometry. This is an interesting finding, as mtHSP70 is a key player in the classic mitochondrial importation pathway [32] . To verify this result, immunoprecipitation using anti-ErbB2 antibody followed by western blotting with mtHSP70, and reverse immunoprecipitation using anti-mtHSP70 antibody followed by western blotting with ErbB2 were performed to determine whether ErbB2 associates with mtHSP70 in MDA-MB-231/ErbB2 cells, which express exogenous ErbB2 ( Fig. 2c , upper). The results showed that both proteins can be detected by western blotting when mitochondrial proteins were immunoprecipitated with antibodies against the other protein. Similar results were obtained with SKBR3 cells ( Fig. 2c , lower). To further confirm that ErbB2 translocates into mitochondria through mtHSP70 pathway, we transfected a siRNA specific to mtHSP70 into SKBR3 cells to knockdown mtHSP70 and examined the distribution of ErbB2 in the cells by western blotting. Figure 2d shows that compared with that of the control scramble siRNA-transfected cells, the amount of ErbB2 in mitochondria was decreased, whereas a relatively larger amount of ErbB2 accumulated in cytoplasm was found in the mtHSP70 siRNA-transfected cells. In contrast, the protein levels of cytochrome c oxidase subunit II in mitochondria were not affected by mtHSP70 knockdown, as this protein is encoded and synthesized in mitochondria and does not participate in the mitochondrial protein importation [33] . Similar results were observed when we transfected SKBR3 cells with another independent siRNA to mtHSP70 ( Supplementary Fig. S4 ). Thus, these data clearly indicate that ErbB2 translocates into mitochondria through an mtHSP70-mediated mitochondrial importation pathway. MtErbB2 switches cancer cell metabolism To examine whether mtErbB2 modulates mitochondrial functions, we transfected the expression vectors containing wild-type ErbB2 (ErbB2WT) and ErbB2 fused to a MTS derived from the mitochondrial electron transfer system (ETS) complex IV (ErbB2Mito) into MDA-MB-231 cells. We also constructed the expression vector containing the aa 623–689 deletion of ErbB2 (ErbB2ΔMTS) and expressed the plasmids in MDA-MB-231 cells. Although the expression of ErbB2 in the whole-cell lysates was similar in 231ErbB2WT, 231ErbB2Mito and 231ErbB2ΔMTS cells, the mtErbB2 expression level in ErbB2Mito cells was much higher than that in ErbB2WT cells (~20-fold measured by protein band intensity quantitation), whereas there was no detectable ErbB2 found in the mitochondrial fraction of 231ErbB2ΔMTS cells, indicating that the MTS signal targets ErbB2 into mitochondria ( Fig. 3a ). To exclude the possibility that transfection might affect mitochondrial integrity, we measured the protein expression of several components of the ETS complexes, including complex I subunit NDUFB8, complex II subunit I p (30 kD), complex III subunit core 2, COX II (cytochrome c oxidase-II) and ATP Synthase F1α in these cells by immunoblotting. All these proteins were expressed in similar amounts in these cells ( Supplementary Fig. S5A ). In addition, the mitochondrial structure and mass of these transfectants were similar as shown by fluorescent microscopy ( Supplementary Fig. S5B ). The amounts of mitochondrial DNA-encoded genes ND1, COX 1, COX 2 and ATP synthase also were similar in these cells measured by real-time quantitative PCR ( Supplementary Fig. S5C ). These results indicate that mitochondrial integrity was not affected by transfection of the ErbB2 expression vectors. 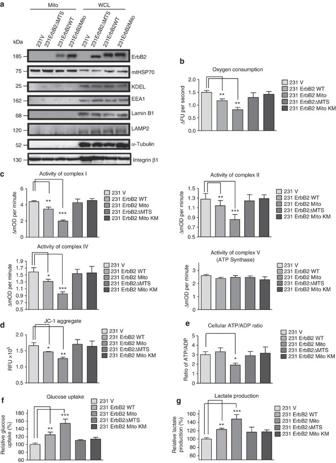Figure 3: MtErbB2 reprograms cellular metabolism from oxidative phosphorylation towards glycolysis. (a) Mitochondrial and whole-cell lysate of 231V, 231ErbB2WT, 231ErbB2Mito, and 231ErbB2ΔMTS cells were isolated and analysed by western blotting. Protein amounts of each fraction loaded: mitochondria: 10 μg; whole-cell lysate: 30 μg. Integrin β1 was used as plasma membrane maker and loading control; mtHSP70 was a mitochondrial maker and loading control; α-tubulin was a cytoplasm maker; KDEL was an ER marker; EEA1 was an early endosomes marker; LAMP2 was an lysosome marker and Lamin B1 was a nucleus marker. (b) Oxygen consumption rates. Oxygen consumption rates of 231V, 231ErbB2WT, 231ErbB2Mito, 231ErbB2ΔMTS and 231ErbB2MitoKM cells were measured. The oxygen consumption rate was calculated on the basis of the maximal rate of change in relative fluorescence units (ΔFU per second). (c) Activities of the mitochondrial electron transport chain complexes in 231V, 231ErbB2WT, 231ErbB2Mito, 231ErbB2ΔMTS and 231ErbB2MitoKM cells. Activities are presented as milliunits of OD value per minute and were normalized by the amounts of the mitochondrial proteins. (d) Mitochondrial membrane potential (Δψm) of 231V, 231ErbB2WT, 231ErbB2Mito, 231ErbB2ΔMTS and 231ErbB2MitoKM cells was detected using JC-1 staining. The aggregate form of JC-1 staining represents healthy mitochondria. (e) The cellular ATP/ADP ratio of 231V, 231ErbB2WT, 231ErbB2Mito, 231ErbB2ΔMTS and 231ErbB2MitoKM cells were detected. (f) MtErbB2 increased glucose uptake. 231V, 231ErbB2WT, 231ErbB2Mito, 231ErbB2ΔMTS and 231ErbB2MitoKM cells were cultured in medium containing 10% fetal bovine serum (FBS) and the glucose uptake were measured. Data are shown as a percentage relative to MDA-MB-231V. (g) MtErbB2 increased lactate production. 231V, 231ErbB2WT, 231ErbB2Mito, 231ErbB2ΔMTS and 231ErbB2MitoKM cells were cultured in medium containing 10% FBS and the lactate production in the medium was measured. Data are shown as a percentage relative to 231V. Columns, mean of three independent experiments; bars, s.e. *P<0.05, **P<0.01, ***P<0.001. Figure 3: MtErbB2 reprograms cellular metabolism from oxidative phosphorylation towards glycolysis. ( a ) Mitochondrial and whole-cell lysate of 231V, 231ErbB2WT, 231ErbB2Mito, and 231ErbB2ΔMTS cells were isolated and analysed by western blotting. Protein amounts of each fraction loaded: mitochondria: 10 μg; whole-cell lysate: 30 μg. Integrin β1 was used as plasma membrane maker and loading control; mtHSP70 was a mitochondrial maker and loading control; α-tubulin was a cytoplasm maker; KDEL was an ER marker; EEA1 was an early endosomes marker; LAMP2 was an lysosome marker and Lamin B1 was a nucleus marker. ( b ) Oxygen consumption rates. Oxygen consumption rates of 231V, 231ErbB2WT, 231ErbB2Mito, 231ErbB2ΔMTS and 231ErbB2MitoKM cells were measured. The oxygen consumption rate was calculated on the basis of the maximal rate of change in relative fluorescence units (ΔFU per second). ( c ) Activities of the mitochondrial electron transport chain complexes in 231V, 231ErbB2WT, 231ErbB2Mito, 231ErbB2ΔMTS and 231ErbB2MitoKM cells. Activities are presented as milliunits of OD value per minute and were normalized by the amounts of the mitochondrial proteins. ( d ) Mitochondrial membrane potential (Δψm) of 231V, 231ErbB2WT, 231ErbB2Mito, 231ErbB2ΔMTS and 231ErbB2MitoKM cells was detected using JC-1 staining. The aggregate form of JC-1 staining represents healthy mitochondria. ( e ) The cellular ATP/ADP ratio of 231V, 231ErbB2WT, 231ErbB2Mito, 231ErbB2ΔMTS and 231ErbB2MitoKM cells were detected. ( f ) MtErbB2 increased glucose uptake. 231V, 231ErbB2WT, 231ErbB2Mito, 231ErbB2ΔMTS and 231ErbB2MitoKM cells were cultured in medium containing 10% fetal bovine serum (FBS) and the glucose uptake were measured. Data are shown as a percentage relative to MDA-MB-231V. ( g ) MtErbB2 increased lactate production. 231V, 231ErbB2WT, 231ErbB2Mito, 231ErbB2ΔMTS and 231ErbB2MitoKM cells were cultured in medium containing 10% FBS and the lactate production in the medium was measured. Data are shown as a percentage relative to 231V. Columns, mean of three independent experiments; bars, s.e. * P <0.05, ** P <0.01, *** P <0.001. Full size image To examine whether mtErbB2 affects the respiratory function of mitochondria, we first measured oxygen consumption, which is a direct indicator of mitochondrial respiration. Oxygen consumption in 231ErbB2Mito cells was decreased compared with 231V and 231ErbB2WT cells ( Fig. 3b ), whereas 231ErbB2ΔMTS cells and kinase-defective mutant ErbB2-transfected cells (231ErbB2MitoKM) had no significant changes, indicating that the overall level of cellular respiration was suppressed by the mitochondrial localization of ErbB2 and the kinase activity of mtErbB2 is required for this. We next conducted assays to examine the enzyme activities of ETS complex I, II, IV and V (ATP synthase). We found that although the proteins were expressed at similar levels ( Supplementary Fig. S5A ), the activities of complex I, II and IV were decreased by mtErbB2. However, the activity of complex V did not change ( Fig. 3c ). We next examined the mitochondrial membrane potential (Δψm), which reflects the efficiency of pumping of hydrogen ions across the inner membrane during the process of electron transport and oxidative phosphorylation, by detecting the aggregation of JC-1 in these cells [31] . We found that the mitochondrial membrane potential of 231ErbB2WT was lower than that of 231V, while 231ErbB2Mito was the lowest and 231ErbB2ΔMTS and 231ErbB2MitoKM cells had no significant changes ( Fig. 3d ). To test whether mitochondrial membrane potential changes resulted in cellular ATP level fluctuation, we measured ATP/ADP levels. The results showed that 231V, 231ErbB2WT, 231ErbB2ΔMTS and 231ErbB2MitoKM cells had a similar ATP/ADP ratio, whereas the ratio in 231ErbB2Mito cells was decreased ( Fig. 3e ). These results clearly indicate that mitochondrial localization of kinase-intact ErbB2 negatively regulates the mitochondrial respiration and oxidative phosphorylation by suppressing the activities of ETS complexes. As glycolysis and mitochondrial oxidative phosphorylation are linked processes [34] , we reasoned that mtErbB2 may increase glycolysis in these cells. To test this, we compared glucose uptake and lactate production, two hallmarks of glycolysis, in 231V, 231ErbB2WT, 231ErbB2Mito, 231ErbB2ΔMTS and 231ErbB2MitoKM cells. We observed that 231ErbB2Mito cells show the highest rates of glucose uptake and lactate production among these cells ( Fig. 3f ), indicating that mtErbB2 promotes glycolysis. Taken together, these results indicate that mtErbB2 switches cancer cell metabolism from oxidative phosphorylation towards glycolysis. MtErbB2 promotes resistance to hypoxia and ETS inhibitors To evaluate whether mtErbB2 causes functional changes in response to cell stress, we treated the cells with specific inhibitors of mitochondrial ETS complexes and glycolysis. We found that mtErbB2 renders cancer cells resistant to the ETS inhibitor oligomycin ( Fig. 4a ), suggesting that 231ErbB2Mito cells are less dependent upon energy supplied by oxidative phosphorylation. In contrast, 231ErbB2Mito cells were more sensitive to the glycolysis inhibitors 2-DG and oxamate, indicating these cells are dependent more upon glycolysis ( Fig. 4a ). These findings are consistent with the results that mtErbB2 negatively regulates cancer cell mitochondrial respiratory functions and promotes glycolysis. We next mimicked a hypoxia environment with CoCl 2 treatment and examined glycolysis indicators in these cells. The results showed that the oxygen consumption of 231V, 231ErbB2WT, 231ErbB2ΔMTS and 231ErbB2MitoKM cells decreased by about 15–30%, whereas 231ErbB2Mito cells were insensitive to hypoxia ( Fig. 4c ). We also observed that under hypoxia, the glucose uptake and lactate production of 231V, 231ErbB2ΔMTS and 231ErbB2MitoKM cells were sharply increased, approaching the levels of the 231ErbB2WT and 231ErbB2Mito cells ( Fig. 4c ), indicating that in a low-oxygen environment, mtErbB2 renders cancer cell less dependent upon the energy supplied by oxidative phosphorylation. 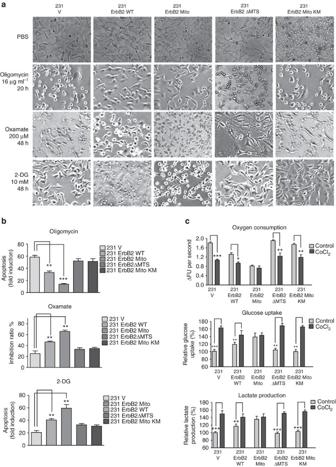Figure 4: MtErbB2 renders cancer cells sensitive to glycolysis inhibitors but resistant to hypoxia and ETS inhibitors. (a) 231V, 231ErbB2WT, 231ErbB2Mito, 231ErbB2ΔMTS and 231ErbB2MitoKM cells were treated with oligomycin at 16 μg ml−1for 20 h; oxamate at 20 μM for 48 h; 2-DG at 10 mM for 48 h and PBS as control. Morphological changes were observed using a microscope (X200). (b) Indicated cells were treated with oligomycin at 16 μg ml−1for 22 h; oxamate at 20 μM for 48 h and 2-DG at 10 mM for 48 h. Direct cell counting was conducted for oxamate treatment. Apoptosis for oligomycin and 2-DG treatments was detected using the Cell Death Detection ELISA PLUS Kit. The fold induction value was calculated following the formula: mU of the sample (cells treated) per mU of the corresponding negative control (cells without treatment). (c) Oxygen consumption rates of non-treated and CoCl2-treated 231V, 231ErbB2WT, 231ErbB2Mito, 231ErbB2ΔMTS and 231ErbB2MitoKM cells. The oxygen consumption rate was calculated on the basis of the maximal rate of change in relative fluorescence units (ΔFU per second) (top). Cells were cultured in medium containing 10% fetal bovine serum, glucose uptake (middle) and lactate production (bottom) of non-treated and CoCl2-treated cells were measured. Data are shown as a percentage relative to 231V cells. Columns, mean of three independent experiments; bars, s.e. *P<0.05, **P<0.01, ***P<0.001. Figure 4: MtErbB2 renders cancer cells sensitive to glycolysis inhibitors but resistant to hypoxia and ETS inhibitors. ( a ) 231V, 231ErbB2WT, 231ErbB2Mito, 231ErbB2ΔMTS and 231ErbB2MitoKM cells were treated with oligomycin at 16 μg ml −1 for 20 h; oxamate at 20 μM for 48 h; 2-DG at 10 mM for 48 h and PBS as control. Morphological changes were observed using a microscope (X200). ( b ) Indicated cells were treated with oligomycin at 16 μg ml −1 for 22 h; oxamate at 20 μM for 48 h and 2-DG at 10 mM for 48 h. Direct cell counting was conducted for oxamate treatment. Apoptosis for oligomycin and 2-DG treatments was detected using the Cell Death Detection ELISA PLUS Kit. The fold induction value was calculated following the formula: mU of the sample (cells treated) per mU of the corresponding negative control (cells without treatment). ( c ) Oxygen consumption rates of non-treated and CoCl 2 -treated 231V, 231ErbB2WT, 231ErbB2Mito, 231ErbB2ΔMTS and 231ErbB2MitoKM cells. The oxygen consumption rate was calculated on the basis of the maximal rate of change in relative fluorescence units (ΔFU per second) (top). Cells were cultured in medium containing 10% fetal bovine serum, glucose uptake (middle) and lactate production (bottom) of non-treated and CoCl 2 -treated cells were measured. Data are shown as a percentage relative to 231V cells. Columns, mean of three independent experiments; bars, s.e. * P <0.05, ** P <0.01, *** P <0.001. Full size image mtErbB2 increases cancer cell trastuzumab resistance Trastuzumab (Herceptin) is a humanized monoclonal antibody, which specifically targets the extracellular domain of ErbB2 and has shown remarkable clinical efficacy in the treatment of ErbB2-positive cancer patients. However, many patients eventually develop resistance to trastuzumab after continuous treatment. The mechanisms of this resistance have been extensively studied, yet the precise mechanism remains elusive. It has been shown that treatment with trastuzumab induces ErbB2 internalization through endocytosis. However, not all the ErbB2 withdrawn from the plasma membrane enters into endosomes and lysosomes ready for degradation [35] . In addition, dysregulated cellular metabolism has been reported to cause cancer cell drug resistance [12] , [13] . Thus, we hypothesized that the treatment of trastuzumab would induce the translocation of the surface-bound ErbB2 into mitochondria and alter cellular metabolism, which may provide a mechanism for trastuzumab resistance. Indeed, we observed a dramatic elevation of mtErbB2 in trastuzumab-resistant cells than that of parental BT474 cells by western blotting ( Fig. 5a ). Trastuzumab induced the translocation of ErbB2 into mitochondria in a time-dependent manner in BT474 cells ( Fig. 5b ; Supplementary Fig. S6A ), whereas the total ErbB2 levels in the cells did not significantly change ( Fig. 5b , right). We next explored whether mtErbB2-overexpressing cells are more resistant to trastuzumab. 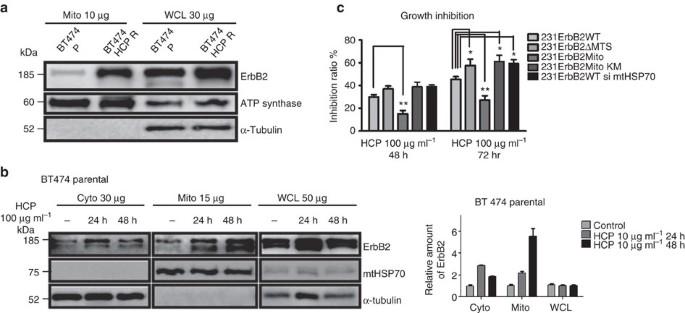Figure 5: Translocation of ErbB2 into mitochondria contributes to trastuzumab resistance. (a) mtErbB2 is elevated in trastuzumab-resistant cancer cells. Mitochondrial proteins and whole-cell lysates of BT474 and BT474 trastuzumab-resistant cells (BT474 HCPR) were isolated and analysed by western blotting. ATP synthase and α-tubulin were used as loading controls. (b) BT474 cells were treated with trastuzumab (HCP) at 10 μg ml−1for 24 and 48 h followed by the separation of cytosolic and mitochondrial fractions. Proteins from the cytoplasm, mitochondria and whole-cell lysates were loaded onto gels and analysed by western blotting. mtHSP70 and α-tubulin were used as loading controls (left). The relative protein amount of ErbB2 in the cellular fractions was calculated by detecting the intensity of the protein bands followed by normalization with loading controls (right). The experiments were repeated for three times. (c) mtErbB2-overexpressing cells are more resistant to trastuzumab. 231ErbB2WT, 231ErbB2Mito, 231ErbB2ΔMTS, 231ErbB2MitoKM and 231ErbB2WT cells transfected by siRNA to mtHSP70 were treated with trastuzumab at 100 μg ml−1for 48 and 72 h. The cell growth inhibition ratios were detected by a CellTiter 96 Aqueous One Solution Cell Proliferation Assay Kit. Columns, mean of three independent experiments; bars, s.e. *P<0.05, **P<0.01. Figure 5c shows that when the cells were treated with 100 μg ml −1 trastuzumab, 231ErbB2Mito cells were more resistant to trastuzumab compared with 231ErbB2WT, 231ErbB2ΔMTS, 231ErbB2MitoKM and 231ErbB2WT cells treated with siRNA to mtHSP70. Importantly, blocking ErbB2 translocation into mitochondria by the deletion of endogenous MTS renders 231ErbB2ΔMTS cells more sensitive to trastuzumab compared with 231ErbB2WT ( P <0.05) and 231ErbB2Mito cells ( P <0.01), indicating that translocation of ErbB2 into mitochondria leads to cancer cell resistant to trastuzumab. These results reveal a novel mechanism for trastuzumab resistance in ErbB2-positive cancer cells. Figure 5: Translocation of ErbB2 into mitochondria contributes to trastuzumab resistance. ( a ) mtErbB2 is elevated in trastuzumab-resistant cancer cells. Mitochondrial proteins and whole-cell lysates of BT474 and BT474 trastuzumab-resistant cells (BT474 HCPR) were isolated and analysed by western blotting. ATP synthase and α-tubulin were used as loading controls. ( b ) BT474 cells were treated with trastuzumab (HCP) at 10 μg ml −1 for 24 and 48 h followed by the separation of cytosolic and mitochondrial fractions. Proteins from the cytoplasm, mitochondria and whole-cell lysates were loaded onto gels and analysed by western blotting. mtHSP70 and α-tubulin were used as loading controls (left). The relative protein amount of ErbB2 in the cellular fractions was calculated by detecting the intensity of the protein bands followed by normalization with loading controls (right). The experiments were repeated for three times. ( c ) mtErbB2-overexpressing cells are more resistant to trastuzumab. 231ErbB2WT, 231ErbB2Mito, 231ErbB2ΔMTS, 231ErbB2MitoKM and 231ErbB2WT cells transfected by siRNA to mtHSP70 were treated with trastuzumab at 100 μg ml −1 for 48 and 72 h. The cell growth inhibition ratios were detected by a CellTiter 96 Aqueous One Solution Cell Proliferation Assay Kit. Columns, mean of three independent experiments; bars, s.e. * P <0.05, ** P <0.01. Full size image Translocation of ErbB2 into mitochondria is kinase dependent As ErbB2 is a receptor tyrosine kinase, we wondered whether the kinase activity of ErbB2 is responsible for the translocation of ErbB2 into mitochondria. We compared the mtErbB2 in multiple MDA-MB-435 variants that express ErbB2 mutants with different tyrosine kinase activities. The 435eb expresses wild-type ErbB2 (435eb), 435V659E (435VE) mutant has an enhanced kinase activity of ErbB2 and 435K753M (435KM) has one amino-acid mutation within the kinase domain, showing a defective kinase activity [36] . The results showed that the expression of mtErbB2 in 435VE cells was much higher than 435eb, whereas the amount of mtErbB2 in 435K753M was the lowest ( Fig. 6a ). To further verify these results, we treated MCF7/ErbB2 cells with Heregulin β1 (HRG), which stimulates the dimerizaiton and activation of ErbB2 or the specific ErbB2 inhibitor AG825, which represses the kinase activity of ErbB2. Compared with those of untreated cells, MCF7/ErbB2 cells exhibited higher mtErbB2 levels when treated with HRG but decreased mtErbB2 when treated with AG825 ( Fig. 6b , upper). HRG indeed increased the phosphorylation of ErbB2, while the treatment with AG825 decreased the phosphorylation although the total amount of ErbB2 in the cells was similar ( Fig. 6b , lower). Similar results were also obtained from the MCF7 cell line, which expresses a moderate ErbB2 level. Similarly, treatment of MCF7 cells with HRG also led to an increased translocation of ErbB2 into mitochondria ( Fig. 6c ). We further confirmed the results by examining the activities of mtErbB2 upon trastuzumab (HCP) treatment on BT474 HCPR trastuzumab-resistant cells. As shown in Supplementary Fig. S7 , in trastuzumab-resistant BT474 HCPR cells, HRG-induced phosphorylation of mtErbB2 was not significantly inhibited by trastuzumab. This result is consistent with our previous results that translocation of ErbB2 into mitochondria is dependent on its kinase activity, which contributes to the function of mtErbB2 in regulating cellular metabolism. 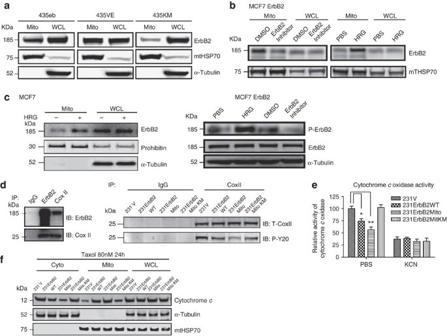Figure 6: Translocation of ErbB2 into mitochondria is kinase dependent. (a) The mitochondrial fractions and whole-cell lysates were isolated and western blotting was performed on MDA-MB-435ErbB2 (435eb), MDA-MB-435ErbB2V695E (435VE) and MDA-MB-435ErbB2K753M (435KM) cells. MtHSP70 and α-tubulin were loading controls. (b) Mitochondrial fractions and whole-cell lysates were isolated and western blotting was performed to detect mtErbB2 in mitochondria following the treatment of MCF7ErbB2 cells with ErbB2 inhibitor AG825 at 10 μM or control (DMSO) for 24 h; and with Heregulin β1 (HRG) at 10 ng ml−1or control (PBS) for 24 h (upper). Whole-cell lysates were subjected to western blotting to examine the phosphorylation status of ErbB2 and the total ErbB2. α-Tubulin was loading control (lower). (c) MCF7 cells were treated with and without HRG at 10 ng ml−1for 24 h. The mitochondrial fraction and the whole-cell lysate were isolated for western blotting. Prohibitin and α-tubulin were loading controls. (d) Left, mitochondrial proteins were isolated from SKBR3 cells and immunoprecipitated with anti-ErbB2 or anti-Cox II antibodies. The immunoprecipitates were analysed by western blotting with anti-ErbB2 and anti-Cox II antibodies. IgG was negative control. Right, mitochondrial proteins were isolated from 231V, 231ErbB2WT, 231ErbB2Mito and 231ErbB2MitoKM cells and immunoprecipitated with Cox II antibody or negative control IgG. Samples were loaded on SDS–PAGE followed by western blotting analysis with Cox II antibody to show the Cox II protein level, and with P-Y20 antibody to show the tyrosine phosphorylation level on Cox II. (e) Cytochromecoxidase activities were measured after the cells were treated with or without a cytochromecoxidase inhibitor potassium cyanide (KCN) in 231V, 231ErbB2WT, 231ErbB2Mito and 231ErbB2MitoKM cells. The relative activities of Cox II were calculated relative to the Cox II activity of 231V cells. (f) 231V, 231ErbB2WT, 231ErbB2Mito and 231ErbB2MitoKM cells were treated with or without Taxol at 80 nM for 24 h. Cytosolic, mitochondrial fractions and whole-cell lysates were analysed by western blotting with cytochromecantibodies. α-Tubulin and mtHSP70 were cytosol and mitochondrial markers and loading controls. Columns, mean of three independent experiments; bars, s.e. *P<0.05, **P<0.01. IP, immunopreciptation; IB, immunoblotting. Figure 6: Translocation of ErbB2 into mitochondria is kinase dependent. ( a ) The mitochondrial fractions and whole-cell lysates were isolated and western blotting was performed on MDA-MB-435ErbB2 (435eb), MDA-MB-435ErbB2V695E (435VE) and MDA-MB-435ErbB2K753M (435KM) cells. MtHSP70 and α-tubulin were loading controls. ( b ) Mitochondrial fractions and whole-cell lysates were isolated and western blotting was performed to detect mtErbB2 in mitochondria following the treatment of MCF7ErbB2 cells with ErbB2 inhibitor AG825 at 10 μM or control (DMSO) for 24 h; and with Heregulin β1 (HRG) at 10 ng ml −1 or control (PBS) for 24 h (upper). Whole-cell lysates were subjected to western blotting to examine the phosphorylation status of ErbB2 and the total ErbB2. α-Tubulin was loading control (lower). ( c ) MCF7 cells were treated with and without HRG at 10 ng ml −1 for 24 h. The mitochondrial fraction and the whole-cell lysate were isolated for western blotting. Prohibitin and α-tubulin were loading controls. ( d ) Left, mitochondrial proteins were isolated from SKBR3 cells and immunoprecipitated with anti-ErbB2 or anti-Cox II antibodies. The immunoprecipitates were analysed by western blotting with anti-ErbB2 and anti-Cox II antibodies. IgG was negative control. Right, mitochondrial proteins were isolated from 231V, 231ErbB2WT, 231ErbB2Mito and 231ErbB2MitoKM cells and immunoprecipitated with Cox II antibody or negative control IgG. Samples were loaded on SDS–PAGE followed by western blotting analysis with Cox II antibody to show the Cox II protein level, and with P-Y20 antibody to show the tyrosine phosphorylation level on Cox II. ( e ) Cytochrome c oxidase activities were measured after the cells were treated with or without a cytochrome c oxidase inhibitor potassium cyanide (KCN) in 231V, 231ErbB2WT, 231ErbB2Mito and 231ErbB2MitoKM cells. The relative activities of Cox II were calculated relative to the Cox II activity of 231V cells. ( f ) 231V, 231ErbB2WT, 231ErbB2Mito and 231ErbB2MitoKM cells were treated with or without Taxol at 80 nM for 24 h. Cytosolic, mitochondrial fractions and whole-cell lysates were analysed by western blotting with cytochrome c antibodies. α-Tubulin and mtHSP70 were cytosol and mitochondrial markers and loading controls. Columns, mean of three independent experiments; bars, s.e. * P <0.05, ** P <0.01. IP, immunopreciptation; IB, immunoblotting. Full size image We next explored mitochondrial proteins that may interact with mtErbB2 and potential substrates of mtErbB2 tyrosine kinase. We isolated mitochondrial fractions from SKBR3 cells and performed immunoprecipitation with antibodies against ErbB2. An SDS–PAGE gel of the immunoprecipitated proteins was stained with Coomassie Blue. The proteins extracted from the gel were subjected to mass spectrometry (data not shown). We found that cytochrome c oxidase-II (Cox II) was among the putative binding partners of mtErbB2. To verify this result, immunoprecipitations using anti-ErbB2 antibody followed by western blotting with Cox II, and reverse immunoprecipitations using anti-Cox II antibody followed by western blotting with ErbB2 were performed to determine whether ErbB2 associates with Cox II in SKBR3 cells. Figure 6d (left) shows that both proteins could be detected by western blotting when mitochondrial proteins were immunoprecipitated with antibody against the other protein, indicating the interaction between mtErbB2 and Cox II. Moreover, we found that the phosphorylation of Cox II was inversely correlated with the kinase activity of mtErbB2 by comparing the phosphorylation levels on Cox II in different ErbB2 mutants-transfected MDA-MB-231 cells ( Fig. 6d , right), suggesting that mtErbB2 regulates the level of tyrosine phosphorylation on Cox II through an indirect mechanism. As phosphorylation on Cox II activates cytochrome c oxidase, which leads to cytochrome c oxidation and to be released from mitochondria to trigger apoptosis [11] , [37] , we compared the cytochrome c oxidase activity among vector alone, ErbB2WT, ErbB2Mito and ErbB2MitoKM cells, as previously described [11] . We found that mitochondrial localization of ErbB2 markedly decreased the activity of cytochrome c oxidase in an ErbB2 kinase-dependent manner ( Fig. 6e ). To examine whether mitochondrial localization of ErbB2 antagonizes apoptosis of cancer cells, we measured cytochrome c release from mitochondria into cytoplasm in these cell variants. 231V, 231ErbB2WT, 231ErbB2Mito and 231ErbB2MitoKM cells were treated with an apoptosis inducer paclitaxel (Taxol), followed by cellular organelle separation and western blotting. 231V and 231ErbB2MitoKM cells are sensitive to Taxol-induced apoptosis, indicated by a significant amount of cytochrome c released from mitochondria into cytoplasm. However, 231ErbB2Mito cells showed the strongest resistance to Taxol with the least releasing of cytochrome c into cytoplasm ( Fig. 6f ), indicating that suppression of Cox II phosphorylation by mtErbB2, which subsequently leads to decreased activity of cytochrome c oxidase, reduced cytochrome c oxidation and less cytochrome c release, contributes to the anti-apoptosis of cancer cells. Recent studies demonstrate that receptor tyrosine kinases can transmit intracellular signals from endosomes and other intracellular compartments, and the precise subcellular location can define signalling specificity in a manner that is not yet understood [38] . Mitochondria have been considered not merely the ‘powerhouses’ of the cell, but also a critical organelle with diverse cellular functions. Mitochondria have crucial roles in apoptosis, reactive oxygen species production and numerous other metabolic processes. Here we report a novel localization of ErbB2 in mitochondria in ErbB2-positive cancer cells and patient samples. This intriguing discovery may open a new avenue for studying the normal and cancerous roles of ErbB2, which may lead to more effective therapeutics for cancer treatment. Moreover, we identified the endogenous MTS of ErbB2 and the association of ErbB2 with mitochondrial transportation protein mtHSP70. Both deletion of the endogenous MTS and downregulation of mtHSP70 blocked the translocation of ErbB2 into mitochondria, suggesting the translocation is physiologically relevant. By immunoprecipitation and mass spectrometry, we validated the interaction of mtErbB2 with Cox II. We observed that the level of phosphorylation on Cox II was inversely correlated with the kinase activity of mtErbB2, suggesting that kinase active mtErbB may activate a phosphatase in mitochondria to de-phosphorylate Cox II. Alternatively, mtErbB2 may lead to de-association of Cox II from a tyrosine kinase that directly phosphorylates Cox II. These results indicate that mtErbB2 may regulate the components of ETS, thus leading to the alteration of mitochondrial function. However, our available data could not exclude the possibility that mtErbB2 regulates mitochondrial respiration through an indirect mechanism. Further investigations are needed on the precise mechanism for how mtErbB2 regulates cancer cell metabolism. It has been reported that EGFR increases glucose uptake independent of its kinase activity [39] . However, we observed that the translocation of ErbB2 into mitochondria is facilitated by ErbB2 tyrosine kinase activation, implying that mtErbB2 phosphorylates substrates in mitochondria to trigger signalling cascades and regulates mitochondrial function. In our previous studies, we found that in breast cancer cells, ErbB2 promotes glycolysis at least partially through the heat shock factor 1 (HSF1)-mediated upregulation of LDH-A [23] . Moreover, trastuzumab inhibits glycolysis via downregulation of HSF1 and LDH-A in ErbB2-positive cancer cells; increased glycolysis contributes to trastuzumab resistance, and targeting glycolysis increases the sensibility of cancer cells to trastuzumab [13] . In the current study, we found that ErbB2 translocates into mitochondria and negatively regulates the respiration function. Collectively, these results suggest that ErbB2 not only promotes glycolysis by upregulating glycolytic enzyme LDH-A but also inhibits mitochondrial oxidative phosphorylation. Both effects of ErbB2 on cellular metabolism drive ErbB2-overexpressing cancer cells towards a Warburg effect-like phenotype. This may explain ErbB2-overexpressing cancer cell’s high capacity to adapt and survive stressful conditions. In summary, our studies demonstrate that a significant amount of ErbB2 is located in mitochondria in cancer cells and patient samples. We found that the translocation of ErbB2 into mitochondria is through a classic mitochondrial translocation pathway facilitated by mtHSP70. Moreover, we found that mtErbB2 regulates mitochondrial respiratory functions and switches the energy dependency of cancer cells from oxidative phosphorylation to aerobic glycolysis. Importantly, we have provided evidence to support that the translocation of ErbB2 into mitochondria is a novel mechanism for trastuzumab resistance. These findings raise important questions such as: what is the detailed mechanism of mtErbB2 regulating the respiratory function of mitochondria? what are the implications of mtErbB2 in cancer development and therapeutics? Answers to these questions will not only solve an intriguing problem for the field of cancer biology but also, more importantly, they may lead to the discovery of a novel biomarker and a therapeutic target for breast and other cancers. Cell lines and cell cultures Human breast cancer cells MCF7, MDA-MB-435, MDA-MB-231, SKBR3, BT474 cells were purchased from the American Type Culture Collection; BT474 and its trastuzumab-resistant variants were gifts from Dr Rita Nahta from Emory University. The cells were cultured in Dulbecco’s modified Eagle’s medium (DMEM)/F-12 (Mediatech Inc., Manassas, VA, USA) with 10% fetal bovine serum in a 5% CO 2 and 37 °C incubator. Antibodies and reagents The antibodies were purchased from: ErbB2 (OP15, Calbiochem), mtHSP70 (MA3-028, Thermo Scientific), VDAC1 (sc-58649, Santa Cruz), Bcl-2 (Rabbit mAb #2870, Cell Signaling), Integrin β (610467, BD Bioscience), prohibitin (EP2803Y, Abcam), KDEL (sc-33806, Santa Cruz), EEA1(sc-130017, Santa Cruz), LAMP2 (sc-18822, Santa Cruz), Lamin B1 (MA1-06103, Thermo Scientific), Mitochondrial Complex I subunit NDUFB8, Complex II subunit 30 kDa, Complex III subunit Core 2, Complex IV subunit II and ATP synthase subunit alpha antibodies mix were MitoProfile Total OXPHOS Human WB Antibody Cocktail (MS601, Mitoscience). siRNAs for mtHSP70(1) (SASI_Hs01_00216924) and mtHSP70(2) (MISSION siRNA SASI_Hs01_00216923) were purchased from Sigma. Protease K was purchased from Sigma; the immunoprecipitation assay was conducted using Pierce Co-immunoprecipitation Kit (Cat: 26149) from Thermo Scientific. Mitotracker was purchased from Invitrogen; intact mitochondria were prepared and purified using Qproteome Mitochondria Isolation Kit from Qiagen; ADP/ATP assay kit was purchased from BioVison; Oxygen Consumption assay kit was from BD Bioscience and Mitochondrial Complex activity assay kits (I, II, IV and V) were purchased from Mitoscience. Mitochondrial membrane potential kit was purchased from BD MitoScreen (JC-1); Glucose uptake was measured using the Amplex Red Glucose/Glucose Oxidase Assay Kit (Molecular Probes, Carlsbad, CA, USA); Lactate production in the medium was detected by using the Lactate Assay Kit (BioVision, Mountain View, CA, USA). Protease K sensitivity Protease sensitivity experiments were conducted with the incubation of intact mitochondria with Proteinase K at 10 μg ml −1 in the presence or absence of 1% Triton-X100. After a 10-min’s incubation at room temperature, reactions were stopped by adding phenylmethylsulfonyl fluoride to a final concentration of 2 mM to stop the reactions. Samples were loaded onto SDS–PAGE and subjected to western blotting analysis. Fluorescence and immunofluorescence microscopy Cells were plated in a 6-well plate on cover glass and cultured overnight. Mitochondria was stained with Mitotracker-Green/Red (Invitrogen) at 100 nM for 30 min, cells were fixed and incubated with primary antibody ErbB2 (mouse) overnight, followed by the incubation of monoclonal mouse Anti-Cy3 antibody (red) or FITC (green). Images were captured with a Nikon Eclipse TE2000-E microscope and were analysed using Nikon NIS-Elements Advanced Research software. Immunotransmission electron microscopy Cancer cells were fixed with 4% paraformaldehyde and 0.1% glutaraldehyde in 100 mM phosphate buffer (PB) (pH 7.4) for 30 min, followed by 1% paraformaldehyde in PB at 4 °C overnight. The samples were then treated in 0.1% sodium borohydride in PB for 15 min, permeabilized with 0.05% Triton-X100 in PB, and blocked with 5% bovine serum albumin (BSA), 0.1% cold water fish skin gelatin and 5% normal goat serum in phosphate-buffered saline (PBS) for 60 min, The primary antibody (mouse anti-ErbB2) incubation was done overnight at 4 °C in PBS containing 0.1% BSA-c. Cells were then rinsed six times with PBS containing 0.1% BSA-c, and incubated with the ultrasmall gold conjugated secondary antibody (Aurion; Wageningen, the Netherlands) in PBS containing 0.1% BSA-c overnight at 4 °C. Afterwards, the samples were rinsed and postfixed with 2% glutaraldehyde followed by rinses with PB and the Enhancement Conditioning Solution (ECS, Aurion). For silver enhancement, sections were agitated in Aurion R-gent SE-EM at room temperature for 2 h and then rinsed in ECS solution again. After additions and rinses in PB, samples were processed and embedded in Epon resin according to standard procedures. Vectors construction Vectors containing wild-type ErbB2 and ErbB2 plus a MTS were constructed. WT-ErbB2 vector was constructed using pEF/myc/cyto vector from Invitrogen. MTS-ErbB2 and MTS-ErbB2-K753M vectors constructed using pEF/myc/mito vector from Invitrogen. The MTS from the pEF/myc/mito is: MSVLTPLLLRGLTGSARRLPVPRAIHSL. Briefly, ErbB2wt and ErbB2 (K753M) CDS were amplified by PCR from plasmids pCDNA3-ErbB2wt or pcDNA3-ErbB2-KD (K753M) with primers: ErbB2 Forward: 5′-TGACTCGAGGAGCTGGCGGCCTTGTGCCGCT-3′; ErbB2 Reverse: 5′-TGAGCGGCCGCCACTGGCACGTCCAGACCCAGG-3′. PCR products were digested with Xho I and Not I and cloned into pEF/myc/cyto or pEF/myc/mito. The pCDNA3-ErbB2wt was amplified by primers to make ErbB2WTΔMTS (deletion of endogenous MTS: 623–689aa): forward primer: 5′-GATGAGGAGGGCGCATGCCTGCAGGAAACGGAGCTG-3′; reverse primer: 5′-CAGCTCCGTTTCCTGCAGGCATGCGCCCTCCTCATC-3′. PCR products were digested with Dpn I and transformed into competitive cells, and MTS deletion was verified by DNA sequencing. Fragments encoding amino acids of ErbB2 juxtamembrane region (aa 646–689), TMD (aa 623–645) and GFP plus TMD fused with juxtamembrane region (aa 623–689) were PCR amplified from pcDNA3-ErbB2wt, cloned between the Eco RI and Bam HI sites of phrGFP-C vector (Stratagene, La Jolla, CA). All constructs were sequenced before use. Plasmid DNA was isolated and transfected into MDA-MB-231 breast cancer cells using Oligofectamin 2000 reagents from Invitrogen in a six-well dish. After 24 h, the cells were transferred into 10 cm dishes containing media (DMEM)/F-12 containing 10% fetal bovine serum and 1.8 mg ml −1 Geneticin. Stable clones were selected and verified by western blotting. Oxygen consumption Oxygen consumption was detected using BD Oxygen Biosensor Systems from BD Bioscience Company. A total of 1 × 10 6 cells were plated into a 96-well plate provided with the kit. The plates were read for fluorescence using the following parameters: 485 nm excitation and 630 nm emission. Raw data was analysed and normalized according to the kit instruction. Each sample was plated in triplicate and each experiment was repeated three times to reach the statistical significance. Mitochondrial complex activity assays The activity of mitochondrial respiration complexes in the electron transfer chain was assayed according to the manufacturer’s protocol using a kit from Mitoscience Company. Specifically, we used mitochondrial Complex I Enzyme Activity Microplate Assay Kit (MS141); Complex II Enzyme Activity Microplate Assay Kit (MS241); Complex IV Human Enzyme Activity Microplate Assay Kit (MS441); ATP synthase Enzyme Activity Microplate Assay Kit (MS541). Briefly, cancer cells, which were stably transfected with ErbB2WT, ErbB2Mito and empty vectors were cultured and total proteins were isolated and subjected to centrifugation at different speeds using lysis buffer/detergents from the kit. The supernatant was incubated in a 96-well microplate with a monoclonal antibody (specific to complex I, II, III and IV accordingly) pre-bound to the wells. After 2–3 h incubation in room temperature, substrates provided from the kit were added into the wells and the absorbance (optical density) was measured in Spectrophotometer for 30 min to 2 h according to the different complex reactions. Raw data was analysed according to the formulas from the protocol. The rate of the reaction was calculated as the complex activity. Glucose uptake assay Cells were seeded in 24-well plates at 5 × 10 5 cells per well. Culture media were collected at 4 and 8 h and stored at −20 °C until assayed. Glucose uptake was measured using the Amplex Red Glucose/Glucose Oxidase Assay Kit (Molecular Probes). Absorbance was measured at 563 nm using a SpectraMax M5 plate reader (Molecular Devices, Sunnyvate, CA, USA) and results were normalized on the basis of the total protein amounts of the cells. Lactate production assay Lactate production in the medium was detected using a Lactate Assay Kit (BioVision). Results were normalized on the basis of the total protein amounts of the cells. Detection of ATP/ADP ratio The ATP/ADP ratios cancer cells were assayed using ApoSENSOR ADP/ATP Ratio Assay Kit from BioVision (Catalog no. K255-200). Cells were cultured and collected. Briefly, 10 μl of the cultured cells (1 × 10 3 –1 × 10 4 ) were transferred into luminometer plate and 100 μl of the Nucleotide Releasing Buffer was added. To measure the ATP levels in the cells, 1 μl of the ATP Monitoring enzyme was added into the cell lysate. The samples were read within 1 min in a luminometer (Data A). To measure ADP levels in the cells, the samples were read after 10 min (Data B) and then 1 μl of ADP Converting enzyme was added. The samples were read again within 1 min in a luminometer (Data C). The ATP/ADP ratio will be calculated as: Data A/(Data C−Data B). Detection of mitochondrial membrane potential Mitochondrial membrane potential was detected using a kit from BD MitoScreen (JC-1) according to the manufacturer’s instruction. MTS prediction MTS was predicted by the online programme: http://psort.ims.u-tokyo.ac.jp/form2.html Cytochrome c oxidase activity assay The cytochrome c oxidase activity assays were performed using the kit from Sigma (CYTOCOX1 cytochrome c oxidase Assay Kit), according to the manufacturer’s instruction. Statistical analysis The unpaired Student’s t -test was used for the data analysis. All data was shown as mean±s.e. A statistical difference of P <0.05 was considered significant. How to cite this article: Ding, Y. et al . Receptor tyrosine kinase ErbB2 translocates into mitochondria and regulates cellular metabolism. Nat. Commun. 3:1271 doi: 10.1038/ncomms2236 (2012).